Membrane tension and peripheral protein density mediate membrane shape transitions Endocytosis is a ubiquitous eukaryotic membrane budding, vesiculation and internalization process fulfilling numerous roles including compensation of membrane area increase after bursts of exocytosis. The mechanism of the coupling between these two processes to enable homeostasis is not well understood. Recently, an ultrafast endocytosis (UFE) pathway was revealed with a speed significantly exceeding classical clathrin-mediated endocytosis (CME). Membrane tension reduction is a potential mechanism by which endocytosis can be rapidly activated at remote sites. Here, we provide experimental evidence for a mechanism whereby membrane tension reduction initiates membrane budding and tubulation mediated by endocytic proteins, such as endophilin A1. We find that shape instabilities occur at well-defined membrane tensions and surface densities of endophilin. From our data, we obtain a membrane shape stability diagram that shows remarkable consistency with a quantitative model. This model applies to all laterally diffusive curvature-coupling proteins and therefore a wide range of endocytic proteins. The cellular processing of signals and cargo is accompanied by the formation of transient, highly curved membrane structures such as tubules and vesicles [1] . One of the best understood membrane transport processes is clathrin-mediated endocytosis (CME). Among other contributors [2] , several types of BAR domain proteins, including endophilin, help induce or stabilize the curvature of clathrin-coated vesicles (CCV) [3] . During clathrin-independent endocytosis, plasma membrane retrieval is modulated by the actions of endophilin and dynamin [4] . Here, we correlate the onset of membrane deformation with the number density of BAR domain proteins on the membrane and evaluate how membrane tension modifies that relationship. Cellular membrane tensions arise from two primary sources: hydrostatic pressure across the lipid bilayer and cytoskeleton–membrane adhesion [5] . These tensions span a range of values from 0.003 mN m −1 to around 0.3 mN m −1 , depending on cell type and state [5] , [6] , [7] . Cells actively maintain their unique membrane tensions and the idea that tension is a regulator of biological processes such as endocytosis has gained attention since the late 1990s [5] , [8] with significantly more contributions in recent years [6] , [9] , [10] , [11] , [12] , [13] , [14] , [15] , [16] , [17] . However, in experiments with biological cells, the magnitude of tension has only been coarsely controlled, if it was controlled at all. We first investigated membrane deformation through the N-terminal BAR domain of endophilin, and then compared these measurements with those obtained with full-length endophilin. To enable tension-controlled measurements, a single micropipette-aspirated giant unilamellar vesicle (GUV, labelled with red fluorophores), consisting of a spherical part and an aspirated part ( Fig. 1a ), was transferred into a solution containing endophilin N-BAR domains (labelled with a green fluorophore) ( Fig. 1b ) [18] . The protein/membrane binding process was quantified by measuring the increase of green fluorescence signal on the GUV contour, which was converted into the molecular density of proteins on the membrane (see Methods) via a calibration method [19] . Simultaneously, the geometry (aspiration length L p and vesicle radius R v , see Fig. 1a ) of the GUV was monitored to document membrane budding/tubulation transitions induced by N-BAR domain binding. Diameters of membrane tubes induced by N-BAR domains are typically below optical resolution [20] , rendering them challenging to image directly, especially during their emergence. However, in our setup, the change in GUV geometry provides a precise indicator for the onset of the membrane shape transition. 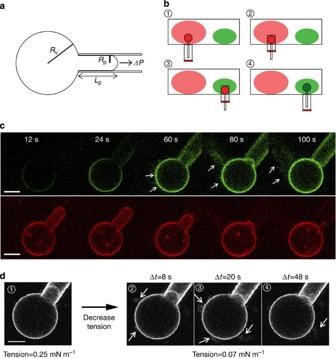Figure 1: Endophilin N-BAR domain induced membrane tubulation of GUV. (a) Sketch of a micropipette-aspirated GUV.ΔPis the pressure difference between inside and outside of the pipette used for GUV aspiration.RpandRvrepresent the pipette radius and the radius of the spherical part of the GUV, respectively,Lprepresents the aspiration length of the GUV. (b) The process of transferring an aspirated GUV from the GUV dispersion (red) into a protein solution (green) (also see Methods). (c) Time lapse confocal images showing the formation of tubes (aftert=24 s, as indicated by arrows) and the change in aspiration length during endophilin N-BAR binding. Membrane tension was held constant at 0.05 mN m−1. Green: protein channel; Red: lipid channel. (d) A GUV incubated to equilibrium with endophilin N-BAR under high tension (0.25 mN m−1). After equilibration, tension was reduced to 0.07 mN m−1within 2 s. Membrane tubes as indicated by arrows can be observed on the GUV under low membrane tension (0.07 mN m−1) forΔtequal to 8 s; 20 s; 48 s (Δt=0 is defined as the time point of tension reduction). Scale bars, 10 μm. Figure 1: Endophilin N-BAR domain induced membrane tubulation of GUV. ( a ) Sketch of a micropipette-aspirated GUV. ΔP is the pressure difference between inside and outside of the pipette used for GUV aspiration. R p and R v represent the pipette radius and the radius of the spherical part of the GUV, respectively, L p represents the aspiration length of the GUV. ( b ) The process of transferring an aspirated GUV from the GUV dispersion (red) into a protein solution (green) (also see Methods). ( c ) Time lapse confocal images showing the formation of tubes (after t =24 s, as indicated by arrows) and the change in aspiration length during endophilin N-BAR binding. Membrane tension was held constant at 0.05 mN m −1 . Green: protein channel; Red: lipid channel. ( d ) A GUV incubated to equilibrium with endophilin N-BAR under high tension (0.25 mN m −1 ). After equilibration, tension was reduced to 0.07 mN m −1 within 2 s. Membrane tubes as indicated by arrows can be observed on the GUV under low membrane tension (0.07 mN m −1 ) for Δt equal to 8 s; 20 s; 48 s ( Δt =0 is defined as the time point of tension reduction). Scale bars, 10 μm. Full size image Effects of protein density and membrane tension When a certain amount of endophilin N-BAR domains was bound on the GUV membrane, the aspiration length L p decreased and membrane tubes grew towards the vesicle exterior until all pipette-aspirated membrane area was consumed (aspiration length L p =0 ) ( Fig. 1c and Supplementary Fig. 1 ). The observed membrane tube formation is consistent with the known capacity of N-BAR proteins to generate membrane curvature [21] . In contrast to the tubulation and corresponding GUV geometry change observed at a membrane tension of 0.05 mN m −1 ( Fig. 1c ), we found that the endophilin N-BAR induced shape instability can be suppressed ( Fig. 1d ) by subjecting vesicles to larger lateral tensions (≥0.25 mN m −1 , see Supplementary Theory ). To investigate how membrane tension affects tubulation, GUVs covered with endophilin N-BAR were subjected to a range of tensions by varying the pipette aspiration pressures. A vesicle under high tension was first equilibrated in the protein chamber to ensure constant coverage of endophilin N-BAR domain, while suppressing tubulation. The tension of the vesicle was then decreased about threefold within 2 s. When the GUV experienced lower membrane tension, membrane tubes emerged around the vesicle, concomitant with a decrease in L p ( Fig. 1d ). Monitoring vesicle radius and aspiration length allows assessing reductions of visible membrane area as growing tubes consume membrane area from the vesicle geometry. Both the protein-induced and tension change-induced membrane tubulations are correlated with a decrease in visible GUV membrane area, as calculated from changes in aspiration length and vesicle radius ( Fig. 2 and Supplementary Fig. 2 , also see Methods). However, besides tubulation, the visible membrane area decrease induced by tension reduction has an additional contribution from entropic membrane fluctuations. We show and discuss in Supplementary Fig. 3 that effects related to membrane fluctuations are substantially smaller than protein effects. 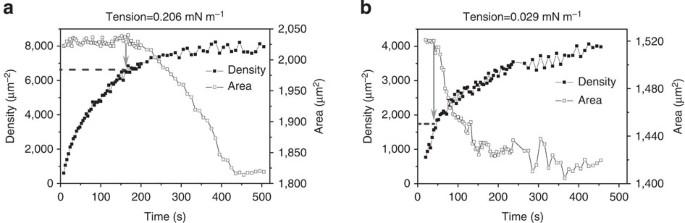Figure 2: Membrane tension and bound protein density modulate membrane shape transition. (a) A representative trial with high (0.206 mN m−1) membrane tension, the membrane-bound endophilin N-BAR density at the onset of area decrease (as indicated by the arrow) genuinely reveals the shape transition point. The area is calculated from the time-dependent aspiration length and vesicle radius as shown inSupplementary Fig. 2b. (b) A representative trial with low (0.029 mN m−1) membrane tension. Transition density (marked by the dashed lines) decreased significantly compared with the high tension case shown ina. Bulk concentrations of endophilin N-BAR are 150 nM inaand 75 nM inb. Potential influence of bulk protein concentration on transition densities was eliminated by comparing the transition densities of similar tension GUVs in endophilin N-BAR solutions of various bulk concentrations (Supplementary Fig. 5a). In addition, there was no observable influence of membrane tension on the endophilin N-BAR’s equilibrium density on GUVs (Supplementary Fig. 5b). Figure 2: Membrane tension and bound protein density modulate membrane shape transition. ( a ) A representative trial with high (0.206 mN m −1 ) membrane tension, the membrane-bound endophilin N-BAR density at the onset of area decrease (as indicated by the arrow) genuinely reveals the shape transition point. The area is calculated from the time-dependent aspiration length and vesicle radius as shown in Supplementary Fig. 2b . ( b ) A representative trial with low (0.029 mN m −1 ) membrane tension. Transition density (marked by the dashed lines) decreased significantly compared with the high tension case shown in a . Bulk concentrations of endophilin N-BAR are 150 nM in a and 75 nM in b . Potential influence of bulk protein concentration on transition densities was eliminated by comparing the transition densities of similar tension GUVs in endophilin N-BAR solutions of various bulk concentrations ( Supplementary Fig. 5a ). In addition, there was no observable influence of membrane tension on the endophilin N-BAR’s equilibrium density on GUVs ( Supplementary Fig. 5b ). Full size image Determining a shape stability diagram To obtain an experimental membrane shape stability diagram correlating protein density and membrane tension at the shape transition, GUVs aspirated at a range of membrane tensions were transferred into endophilin N-BAR solutions ( Fig. 2 ). Potential osmotic contributions to changes in vesicle geometry were carefully excluded ( Supplementary Figs 2 and 4 ). Consistently, we observed formation of membrane tubes, and the associated decrease in visible membrane area, only after the protein density on GUVs reached a well-defined threshold level, indicating the existence of a protein transition density required for inducing membrane tubulation. We define the transition density as the protein density at which visible membrane area of GUVs begins to decrease, as indicated by the arrows in Fig. 2 . The transition density has no observable dependence on the protein concentration in the bulk solution ( Supplementary Fig. 5a ). However, comparison between a high-tension GUV ( Fig. 2a ) and a low-tension GUV ( Fig. 2b ) reveals a striking influence of membrane tension on the transition density with minimal effect on protein–membrane binding ( Supplementary Fig. 5b ). We constructed a membrane shape stability diagram by systematically determining the transition densities of the protein for GUVs under various membrane tensions ( Fig. 3 ). This stability diagram was obtained for GUVs with the composition 1,2-dioleoyl- sn- glycero-3-phospho-L-serine/1,2-dioleoyl- sn -glycero-3-phosphoethanolamine/1,2-dioleoyl-sn-glycero-3-phosphocholine (DOPS/DOPE/DOPC)=45/30/25 with membrane-bound endophilin N-BAR domains. This lipid composition was chosen to mimic the inner leaflet headgroup composition of plasma membranes, where endocytic events take place [22] . Di-oleoyl lipid chains were chosen to suppress lipid demixing. 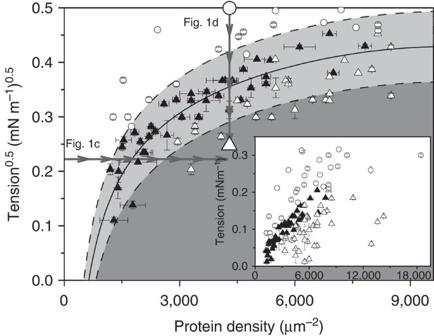Figure 3: Experimental shape stability diagram agrees well with curvature instability theory. Filled triangles represent the measured transition density of protein-covered GUVs under corresponding tensions. The open data points represent the maximum protein density reached by a GUV with (triangle) or without (circle) tubulation during protein–membrane binding. The solid line represents the best fit of experimental data with the proposed curvature instability model (r2=0.85). The dashed lines are 95% confidence intervals for the fit. The shaded area represents the region where the membrane is tubulated by endophilin N-BAR. The arrows indicate two ways of inducing membrane tubulation: (1) by increasing protein coverage on the membrane at constant tension or (2) by decreasing membrane tension at constant coverage. The large circle (non-tubulated state) and triangle (tubulated state) represent the state of the membrane before and after tension reduction (compareFig. 1d), respectively. The inset shows the same data using linear axes. Error bars represent the standard errors associated with determining each data point. Concentrations of endophilin N-BAR used in the experiment ranged from 25 to 400 nM (also noteSupplementary Fig. 5a). Figure 3: Experimental shape stability diagram agrees well with curvature instability theory. Filled triangles represent the measured transition density of protein-covered GUVs under corresponding tensions. The open data points represent the maximum protein density reached by a GUV with (triangle) or without (circle) tubulation during protein–membrane binding. The solid line represents the best fit of experimental data with the proposed curvature instability model ( r 2 =0.85). The dashed lines are 95% confidence intervals for the fit. The shaded area represents the region where the membrane is tubulated by endophilin N-BAR. The arrows indicate two ways of inducing membrane tubulation: (1) by increasing protein coverage on the membrane at constant tension or (2) by decreasing membrane tension at constant coverage. The large circle (non-tubulated state) and triangle (tubulated state) represent the state of the membrane before and after tension reduction (compare Fig. 1d ), respectively. The inset shows the same data using linear axes. Error bars represent the standard errors associated with determining each data point. Concentrations of endophilin N-BAR used in the experiment ranged from 25 to 400 nM (also note Supplementary Fig. 5a ). Full size image We found that full-length endophilin shows a qualitatively similar membrane tubulation behaviour as its N-BAR domain, albeit with higher transition densities compared with the N-BAR domain ( Fig. 4 ), consistent with a potential autoinhibition of endophilin function [23] . 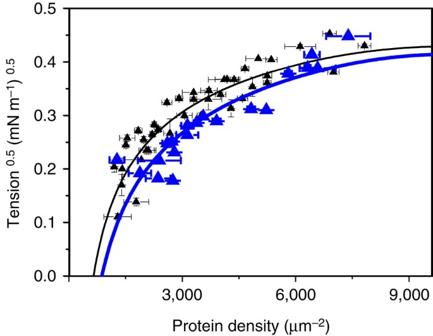Figure 4: Full-length protein shows smaller curvature generation capacity than N-BAR. Transition densities of full-length endophilin (blue triangles), as well as the best fit with our curvature instability model (blue line,r2=0.75) are plotted on top of the stability diagram of N-BAR displayed inFig. 3for GUVs with the same lipid composition (DOPS/DOPE/DOPC=45/30/25). The physical properties resulting from fitting the endophilin full-length data are: the spontaneous curvatureC0−1=6.1±1.1 nm; the upper tension limitσ*=0.17±0.04 mN m−1; the protein transition density required for tubulating a tensionless membraneρ0=850±300 μm−2.P=0.035 between the stability boundaries of endophilin full length and N-BAR viaf-test. Error bars represent the standard errors associated with determining each data point. Figure 4: Full-length protein shows smaller curvature generation capacity than N-BAR. Transition densities of full-length endophilin (blue triangles), as well as the best fit with our curvature instability model (blue line, r 2 =0.75) are plotted on top of the stability diagram of N-BAR displayed in Fig. 3 for GUVs with the same lipid composition (DOPS/DOPE/DOPC=45/30/25). The physical properties resulting from fitting the endophilin full-length data are: the spontaneous curvature C 0 −1 =6.1±1.1 nm; the upper tension limit σ *=0.17±0.04 mN m −1 ; the protein transition density required for tubulating a tensionless membrane ρ 0 =850±300 μm −2 . P =0.035 between the stability boundaries of endophilin full length and N-BAR via f -test. Error bars represent the standard errors associated with determining each data point. Full size image The stability diagram ( Fig. 3 ) illustrates how two factors, density increase (horizontal arrows) and tension decrease (vertical arrows), can be used to control the transformation of lipid membranes from a planar (white) to tubular (dark grey) state. These two trajectories in the stability diagram correspond to the scenarios in Fig. 1c and d respectively. The stability diagram shows a positive intercept ρ 0 of the stability boundary on the x axis (displaying number density of N-BAR dimers on the membrane). This is consistent with the fact that at vanishing membrane tension, GUVs with identical lipid compositions in both leaflets are stable towards tubulation in the absence of curvature-inducing proteins. Analytical model based on three adjustable parameters We next aim to fit a biophysical model to our data, with the goal to illuminate molecular details of the curvature instability induced by endophilin. We seek the following features of a suitable model: (a) it should allow for locally varying protein densities on the membrane in a temperature-dependent manner, to account for entropic contributions to shape stability; (b) it should feature a coupling between local protein density and membrane curvature; (c) the exact geometry of the membrane after deformation does not need to be prescribed by the model, because we focus on the onset of the shape instability. While several theories have been developed to explain the spontaneous budding/tubulation of membranes [24] , [25] , [26] , only the linear stability theory [27] used in the following is consistent with the requirements listed above. Note that the shape of the membrane after undergoing the instability would have to be described with a non-linear approach [28] . Using σ to represent the membrane tension and to represent the average cover fraction of proteins on the membrane (experimentally the cover fraction is obtained by dividing the measured N-BAR dimer density to its close-packed density ρ max =30,000 μm −2 (ref. 29 )), the instability criterion can be written as (see Supplementary Theory for details), Here, κ is the bending rigidity, C 0 describes the spontaneous curvature of the membrane induced by protein binding (positive for N-BAR domains), k B is the Boltzmann constant and the T is the temperature. The parameter b is normally a constant and can be expressed in a simple lattice model as b=λ ( βk B T ) −1 where β is the excluded area of the protein and λ represents an effective ‘interaction area’ for molecular interactions in a protein density gradient [30] . The parameter α represents the attraction strength between protein molecules in the two-dimensional Van der Waals model [31] . It follows from Equation 1 that the experimentally determined stability limit can be fitted with the expression , with a i being parameters that are optimized to yield the best fit with the experimental data. These three fit parameters, a 1 to a 3 , are directly related to three molecular properties of the protein: C 0 , b and α ( Supplementary Equation 11 ). Furthermore, these molecular properties can be correlated with a set of three measurable physical properties: the protein’s membrane curvature-coupling strength: κC 0 , the maximal tension that allows the curvature instability: σ * and the protein density required for tubulating a tensionless membrane: ρ 0 ( Supplementary Equation 12 ). As shown in Fig. 3 , the model is in good agreement with the measured relation between transition density and membrane tension. To be able to obtain the spontaneous curvature from the value of the curvature-coupling strength κC 0 , we measured the bending rigidity of the membrane used here (DOPS/DOPE/DOPC=45/30/25) as κ =23±3 k B T (mean±s.d., repeated for five GUVs, also see Methods and Supplementary Fig. 6 ). Assuming β =50 nm 2 (ref. 19 ), the fit results correspond to a spontaneous curvature C 0 −1 =5.1±0.7 nm (here and where not further specified below, uncertainties result from the standard error of fit parameters and error propagation) agreeing well with values inferred from N-BAR protein curvature sorting experiments performed on a GUV–tether system [19] , [31] . The upper tension limit for enabling membrane shape transitions through endophilin N-BAR for the lipid composition used here is σ *=0.19±0.04 mN m −1 . Finally, the protein transition density required for tubulating a tensionless membrane is ρ 0 =650±150 μm −2 , corresponding to about 7.5 protein dimers on a CCV-sized membrane (assuming a CCV radius of 30 nm). Interestingly, the total number of endophilin molecules in synaptic boutons was measured in a recent study [32] . An endophilin dimer density of 546±36 μm −2 on the synaptosome surface can be estimated (see Supplementary Theory for details). This endophilin density turns out to be within the stable regime of the stability diagram (for any membrane tension), but is localized close to the stability boundary (assuming typical neuronal membrane tensions of 0.003–0.04 mN m −1 (ref. 5 )). This suggests that under physiological conditions, the plasma membrane of neuronal cells can easily switch between stable (endocytosis suppressed) and unstable (endocytosis activated) states by changing membrane tension or locally concentrating proteins such as endophilin. We reiterate in passing that our shape stability theory describes the capacity of a peripheral protein to generate curvature not only with the well-known spontaneous curvature, but with two additional parameters related to molecular details of the protein/membrane system: the protein density for tubulating a tensionless membrane, and the maximal tubulation tension. In future contributions we will demonstrate that these parameters can vary substantially, comparing different types of curvature sensitive peripheral membrane proteins. Shape stability boundary is unaffected by binding kinetics We note that the biophysical shape stability fitted to our experimental data is valid only under thermodynamic equilibrium conditions—an assumption that needs verification. We, therefore, investigated if binding kinetics of proteins to the membrane measurably affects the transition density. Negatively charged phosphatidylserine (PS) lipids can affect the binding kinetics of proteins both in vivo and in vitro [18] , [33] . Specifically, a larger fraction of PS lipids in the membrane is known to increase the membrane binding rate of the endophilin N-BAR domain [18] . To test the thermodynamic equilibrium hypothesis, we measured the membrane shape transition points for vesicles containing different amounts of negatively charged lipids. Not surprisingly, the equilibrium density of proteins on the membrane significantly increases with an increasing amount of PS lipids in GUVs ( Fig. 5 ). Interestingly, however, transition densities, as well as the tension dependence, are identical within uncertainties for the three lipid compositions tested ( Fig. 5 and Supplementary Fig. 7 ). Equivalently, for the same lipid composition, only equilibrium densities, but not transition densities, depend on bulk protein concentration ( Supplementary Fig. 5a ). To further validate the hypothesis that membrane binding kinetics do not affect our results, we measured an apparent protein binding rate by determining the slope of the protein binding curve in a time interval close to the shape instability ( Supplementary Fig. 8a ). Using GUVs under the same membrane tension (0.110±0.007 mN m −1 , mean±s.d. ), we found that transition densities exhibit no dependence on the apparent protein binding rate (see Supplementary Fig. 8b , showing a zero slope within statistical error (7.5±10 s)). We, therefore, conclude that under our conditions, protein–membrane binding kinetics plays a negligible role in controlling the membrane curvature instability. 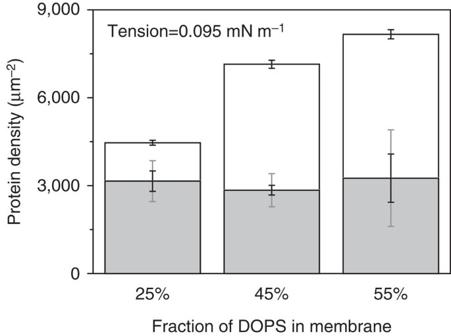Figure 5: Membrane charge affects equilibrium density, not transition density. Equilibrium densities of endophilin N-BAR (open bars) increase significantly for increasing amounts of DOPS in the GUV (for each composition pairP<10−4, Student’st-test). No significant difference can be found among the transition densities (grey bars, for each composition pair,P>0.5, Student’st-test). Concentration of endophilin N-BAR domain: 100 nM. GUV compositions: DOPS/DOPE/DOPC=X/30/(70-X). All GUVs considered here are at the membrane tension of 0.095±0.013 mN m−1(mean±s.d.). Grey error bars are standard deviations (s.d.) of the data and black error bars are standard errors of the mean (s.e.m.), same below. Figure 5: Membrane charge affects equilibrium density, not transition density. Equilibrium densities of endophilin N-BAR (open bars) increase significantly for increasing amounts of DOPS in the GUV (for each composition pair P <10 −4 , Student’s t -test). No significant difference can be found among the transition densities (grey bars, for each composition pair, P >0.5, Student’s t -test). Concentration of endophilin N-BAR domain: 100 nM. GUV compositions: DOPS/DOPE/DOPC=X/30/(70-X). All GUVs considered here are at the membrane tension of 0.095±0.013 mN m −1 (mean±s.d.). Grey error bars are standard deviations (s.d.) of the data and black error bars are standard errors of the mean (s.e.m. ), same below. Full size image Lipid shape as an additional control parameter We finally asked if lipid shape can affect the shape transition density for endophilin N-BAR. 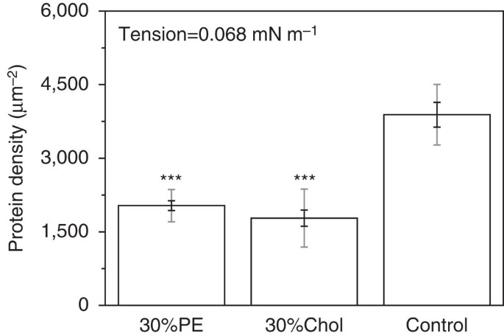Figure 6: The effect of conical lipids on membrane shape transitions. Under the same membrane tension (0.068±0.007 mN m−1(mean±s.d.)), the presence of 30% conical lipids, either DOPE or cholesterol, significantly lowers the transition density of endophilin N-BAR domain. ***P<10−4, Student’st-test. Figure 6 shows that the cone-shaped lipids cholesterol and DOPE both significantly reduce the transition density at constant membrane tension. This amplification effect of cone-shaped lipids on membrane tubulation is consistent with previous observations in a different experimental system [26] . However, only the presence of DOPE but not cholesterol lowers the bending rigidity of the membrane ( Supplementary Fig. 6 ). Therefore, at least for cholesterol, we can attribute its effect on the transition density to the conical lipid shape [34] , [35] . It is well known that proteins with membrane curvature insertion ability will lead to different spontaneous curvature of the membrane depending on the protein’s insertion depth [36] . Therefore, in the presence of conical lipids, the protein’s coupling strength to membrane curvature may be altered by allowing the protein to insert more deeply into the lipid bilayer—a hypothesis that remains to be tested. In addition to membrane tension and protein density, lipid shape provides a third level of control that cells can use to regulate membrane shape transitions ( Fig. 7 ). Figure 6: The effect of conical lipids on membrane shape transitions. Under the same membrane tension (0.068±0.007 mN m −1 (mean±s.d. )), the presence of 30% conical lipids, either DOPE or cholesterol, significantly lowers the transition density of endophilin N-BAR domain. *** P <10 −4 , Student’s t -test. 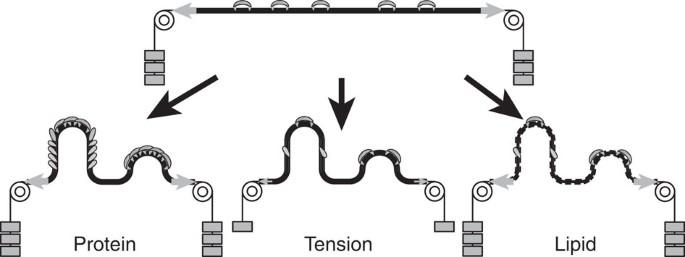Figure 7: Three ways of mediating membrane curvature instability. Three regulatory elements are identified in this contribution that can modulate membrane shape transitions induced by the binding of curvature-coupling proteins. Notably, membrane budding and tubulation is not solely induced by protein association (left arrow). The effects of lowering membrane tension (middle arrow) and changing membrane lipid composition (right arrow) also control membrane shape transition without the assistance of additional proteins. The contribution of peripheral proteins is defined by their density on the membrane, emphasizing a thermodynamic role played by protein molecules in mediating membrane shape transitions. The tension effect may explain an ultrafast pathway cells can utilize to control membrane shape transformations such as endocytosis. Full size image Figure 7: Three ways of mediating membrane curvature instability. Three regulatory elements are identified in this contribution that can modulate membrane shape transitions induced by the binding of curvature-coupling proteins. Notably, membrane budding and tubulation is not solely induced by protein association (left arrow). The effects of lowering membrane tension (middle arrow) and changing membrane lipid composition (right arrow) also control membrane shape transition without the assistance of additional proteins. The contribution of peripheral proteins is defined by their density on the membrane, emphasizing a thermodynamic role played by protein molecules in mediating membrane shape transitions. The tension effect may explain an ultrafast pathway cells can utilize to control membrane shape transformations such as endocytosis. Full size image It has to be emphasized that we have used the simplest thermodynamic theory of membrane stability in the presence of curvature-inducing proteins, which neglects the highly anisotropic spontaneous curvature and significant oligomerization tendency of N-BAR domain proteins [18] , [37] , [38] , [39] , [40] . Nevertheless, our model accurately describes the shape transition. Precisely because the model does not assume details about the protein other than a non-zero curvature-coupling strength and an excluded area for the protein, it likely applies to all endocytic proteins. The presence of a well-defined membrane shape transition density provides an attractive explanation for how endocytic protein recruitment can control plasma membrane deformation during CME: the initiation of membrane buds and the formation of a CCV may proceed only after establishing well-defined transition densities of endocytic proteins. For UFE, however, the endocytic vesicle formation route of a 10 ms duration leaves little time for a plasma membrane patch to undergo a sequential protein recruitment process as in CME (typically 10–20 s (ref. 2 )). Thus, instead of recruiting additional curvature generating proteins to the membrane, for the case of UFE, a more plausible signal that triggers membrane budding is the lowering of membrane tension in the presence of already membrane-bound peripheral proteins. Owing to the membrane fluidity, tension changes propagate at a speed of about 10 6 μm s −1 (refs 11 , 41 ). Therefore, a tension reduction caused by processes such as the fusion of exocytic vesicles into the plasma membrane can likely trigger endocytosis at a much faster rate compared with the process of recruiting peripheral curvature-inducing proteins. For classical endocytosis, a checkpoint that separates abortive from propagating endocytic pits has been identified [42] , [43] . It is possible that the stability boundary identified in our shape diagram provides a mechanistic explanation for this phenomenon. Abortive endocytic pits might assemble owing to local fluctuations in protein density and membrane tension, but in situations where the stability boundary is not passed such fluctuations will eventually decay without producing vesicles. Our findings provide new insights into how cellular membrane shapes and dynamics are controlled by interacting with curvature-coupling proteins, as well as via the regulation of membrane physical properties such as tension and lipid shape. We suggest that the coupling of membrane tension and density of curvature-coupling proteins determined here plays modulatory roles in all forms of endocytosis. Materials Lipids DOPC, DOPS, DOPE, cholesterol (Chol) and distearoylphosphatidylethanolamine-N-(biotinyl(polyethylene glycol)2000) (DSPE-Bio-574 PEG2000) were obtained from Avanti Polar Lipids (Alabaster, AL). Alexa Fluor 488 (AF-488) C5-maleimide, BODIPY FL DHPE (N-(4,4-difluoro-5,7-dimethyl-4-bora-3a,4a-diaza-s-indacene-3-propionyl)-1,2-dihexadecanoyl-sn-glycero-3-phosphoethanolamine, triethylammonium salt) and Texas Red-1,2-dihexadecanoyl-sn-glycero-3 phosphoethanolamine (triethylammonium salt) were from Invitrogen/Life Technologies (Grand Island, NY). Casein, Tris, HEPES and EDTA were obtained from Fisher Scientific (Rochester, NY). All commercial reagents were used without further purification. Streptavidin-conjugated microspheres with mean diameter of ~6 μm were from Polysciences, Inc. (Warrington, PA). An additional 0.5% DSPE-Bio-574 PEG2000 was added into the lipid mixture when preparing GUVs for membrane bending rigidity measurements through tether pulling. Rat endophilin A1 N-BAR_C241 (residues 1–247) and full-length endophilin A1 were expressed, purified and labelled with AF-488 as described [18] , [23] . Protein concentrations were determined by Bradford analysis using bovine serum albumin (Thermo) as a standard. Concentrations indicated refer to total concentration of endophilin in terms of dimeric units. Imaging chamber preparation and GUV transfer procedures GUVs were prepared in 300 mM sucrose solution by the standard method of electroformation with 0.3% Texas Red-DHPE in desired lipid compositions, using indium tin oxide covered glass slides onto which thin films of lipids were prepared from chloroform solutions [44] . Two imaging chambers, GUV chamber and protein chamber, were formed between two coverslips (20 × 40 mm, pre-treated with 2 μl of 2.5 mg ml −1 casein, 20 mM Tris and 2 mM EDTA) overhanging a glass microscope slide (2-mm thick). The GUV chamber has a total volume of 375 μl and is made by diluting 5–8 μl of the GUV stock solutions into a buffer containing glucose, sucrose, NaCl and HEPES. The osmolarity of the buffer was selected to be 20% higher than the GUV stock solution (measured with a micro-osmometer, Advanced Instruments Inc. (Norwood, MA)) to ensure that the vesicles had enough excess area for micropipette aspiration. The protein chamber had a total volume of 187.5 μl. The protein stock solution was diluted to designated concentrations, using the same buffer as used for diluting GUVs. For both the chambers, we chose pH=7 and NaCl was kept at 50 mM, with 7 mM HEPES. Sucrose and glucose (1:1) concentrations were adjusted to yield total osmolarities of the desired values. Micropipettes and transfer capillaries were prepared and casein treated through incubation with saturated casein solutions followed by rinsing [18] , [44] . Occasionally, GUV membranes were observed to stick to pipette walls. Data from such vesicles were discarded. The GUV transfer was a four-step process as shown in Fig. 1b : (1) A GUV was aspirated into a micropipette to adjust the desired membrane tension. (2) The transfer capillary was manually positioned to cover the GUV. (3) The GUV was transferred from the GUV chamber into the protein chamber using a motor-controlled micromanipulator (Luigs and Neumann, Ratingen, Germany). (4) The transfer capillary was removed to expose the GUV to protein. The moment when the GUV was not protected anymore by the transfer capillary was defined as time zero in the protein–GUV association analysis. Zero aspiration pressure was checked before and after the protein–GUV association process to ensure the absence of pressure drifts [45] . All the transfer and imaging processes were carried out at room temperature (23.7±0.3 °C; mean±s.d. measured on different days). Microscopy and data analysis The protein–membrane association process and the membrane geometry changes were monitored with a confocal fluorescence microscope [44] , using a 60 × 1.1 N.A. objective (Olympus, Center Valley, PA). The aspiration length L p , micropipette radius R p and GUV radius R v were measured with Image J, as illustrated in Fig. 1a . The GUV geometry was calculated as area( t )=4 πR v ( t ) 2 +2 πR p L p ( t ), volume( t )=4 πR v (t) 3 /3+ πR p 2 L p ( t ). The average protein fluorescence intensity was determined by fitting a Gaussian ring to the GUV contour (excluding the aspirated region) using MATLAB. R v can also be obtained from the fitting and was checked through a direct measurement via Image J. The measured fluorescence intensity was then converted to protein number density ρ ( t ) on the membrane, using the method of ref. 19 , as follows. GUVs containing x % BODIPY and (100− x )% DOPC were prepared ( x : 0.1–0.7) and at least ten independent GUVs were imaged under the same settings as during the recording of GUV–protein association. A linear fit ( r 2 =0.99) was carried out to get the relation between measured GUV fluorescence intensity and BODIPY density on the membrane. The quantum yield difference between BODIPY and AF-488 was determined to be BODIPY/‘AF-488’=0.5, by imaging bulk solution intensity of SUVs (containing BODIPY) and AF-488-labelled proteins under the same solution conditions as in our experiments (50 mM NaCl, pH 7) [46] . The average lipid headgroup area was assumed as 0.7 nm 2 . The relation between imaged average fluorescence intensity (in arbitrary units for 16-bit images) and dimeric endophilin N-BAR density ( ρ in the unit of μm −2 ) on GUVs is: fluorescence intensity/ labelling efficiency=(4.9±0.2) × ρ . The membrane shape transition point t c was defined as the time point when area( t ) begins to decrease ( Fig. 2 ) and the corresponding protein density ρ ( t c ) was defined as the transition density. Membrane bending rigidity measurements A 1-mm thick sample chamber was formed by overhanging two coverslips on both sides of a microscope glass slide. The bottom of the chamber was pre-treated with 2 μl of 2.5 mg ml −1 casein in 20 mM Tris-HCl and 2 mM EDTA to prevent adhesion of beads and GUVs to the coverslip. The chamber was filled with 1 μl of microsphere dispersion, 5 μl of GUV dispersion and 90–100 μl of the same sucrose, glucose, NaCl and HEPES mixture as described above, resulting a final environment containing 50 mM NaCl. The chamber was mounted on an inverted microscope (1X71; Olympus, Center Valley, PA) equipped with a home built optical trap as described in refs 45 , 46 . A GUV (about 10 μm in radius) was aspirated at a constant pressure and subsequently brought into contact with a trapped bead. Then the bead was moved at 10 μm s −1 to pull out a membrane tether of 20 μm in length. The tether pulling force f is determined as for a Hookean spring: f=kΔx , where k is the trap stiffness and Δx is the displacement of the bead relative to its equilibrium position. The stiffness of the trap with a typical value of 0.05 pN nm −1 was calibrated by the drag force method [47] for multiple beads. Aspiration pressure was changed after the formation of a stable tether to obtain the relation between tether pulling force and membrane lateral tension. Each lateral tension was maintained until the pulling forces reached equilibrium (typically a few seconds). Membrane bending rigidity was subsequently extracted from the relation: (ref. 48 ). For each lipid composition used, force-tension relations and thus bending rigidities were measured on tethers pulled from at least five independent GUVs. How to cite this article: Shi, Z. and Baumgart T. Membrane tension and peripheral protein density mediate membrane shape transitions. Nat. Commun. 6:5974 doi: 10.1038/ncomms6974 (2015).